Evidence of Stranski–Krastanov growth at the initial stage of atmospheric water condensation The precipitation products (rain, snow and so on) of atmospheric water vapour are widely prevalent, and yet the map of its initial stage at a surface is still unclear. Here we investigate the condensation of water vapour occurring in both the hydrophobic–hydrophilic interface (graphene/mica) and the hydrophilic–hydrophilic interface (MoS 2 /mica) by in situ thermally controlled atomic force microscopy. By monitoring the dynamic dewetting/rewetting transitions process, the ice-like water adlayers, at the hydrophobic–hydrophilic interface and not at the hydrophilic–hydrophilic interface, stacked on top of each other up to three ice –I h layers (each of height 3.7±0.2 Å), and the transition from layers to droplets was directly visualized experimentally. Compared with molecular dynamics simulation, the Stranski–Krastanov growth model is better suited to describe the whole water condensation process at the hydrophobic–hydrophilic interface. The initial stage of the hydrometeor is rationalized, which potentially can be utilized for understanding the boundary condition for water transport and the aqueous interfacial chemistry. Hydrometeor (rain, snow and so on) is one of the most common phenomena in nature. Under ambient conditions, most anomalous phases involve water, and the relevant transition on solid surfaces is of fundamental importance [1] . For the past three decades, researchers have successfully revealed the initial arrangement of water molecules as one hexagonal layer of the naturally occurring ice crystal, ‘ice –I h ’, at cryogenic temperatures [2] , [3] . Because water has stronger affinity to surface than to itself, a thin ice bilayer can grow on both hydrophilic and hydrophobic surfaces [4] . Only with accumulation of strain (from mismatch) and electrostatic energy terms (from dipole orientation) could the multilayer growth of water above the first bilayer be observed experimentally [5] . The existence of contamination introduces the relaxation of stress, as a result of which the transition from flat layers to droplets could be explained by the Stranski–Krastanov (SK) mode [4] . These studies benefited from the powerful surface science techniques under vacuum and cryogenic temperature conditions, combined with theoretical calculations [2] . Although the investigations under high-vacuum and cryogenic temperature conditions have revealed the whole process of water vapour condensation, the results cannot be directly applied to water condensation under ambient conditions (1 atm at room temperature (RT)). In particular, previous experiments have suggested that the dipole orientation of the first ice-like bilayer is opposite between below the melting point and above the melting point [6] . In the context of our daily life, it is worthwhile to directly investigate the growth of water adlayers at RT. Scanning probe microscopes [7] , such as the scanning tunnelling microscope and the atomic force microscope (AFM), give detailed insight into the dynamics of molecules and structures with molecular resolution, but remain challenging for imaging free liquid surfaces under ambient conditions. When the probe approaches the liquid surface, strong capillary forces will cause the liquid to wet the tip and will strongly perturb the liquid [8] , [9] . Different non-contact AFM and scanning polarization force microscopy methods have been developed to overcome many of these problems and have provided important results, but a disadvantage is that the large distance between the tip and the sample results in lower spatial resolution. Recently, graphene, albeit only one-atom thick, was found to not only prevent the evaporation of molecularly thin adlayers but also to act as an ideal template for studying the structures of ultrathin liquid adlayers on solid support under ambient conditions [10] , [11] , [12] , [13] , [14] , [15] . With the assistance of graphene, Xu et al. [11] pioneered work on the observation of the first two ice-like water adlayers, increasing the humidity to 90%. Similar phenomena have been reported between the interface of graphene and SiO 2 (hydrophilic substrate) [16] . Both of them have found that the thicknesses of single and double layers of water are the same as that of single and double layers of normal ice (ice –I h ), and suggested that the water can epitaxially grow in a strictly Frank-van der Merwe (FM) manner. However, these experiments are all under high supersaturation condition (up to 90% humidity), which has limitations in providing direct evidence for the detailed growth mechanism and also limits the reflecting of the natural water condensation at ambient conditions. Temperature is one of the key parameters for water transition. Water adlayer growth under temperature control conditions is necessary, especially at nanoscale. An alternate approach is to control the environment temperature in situ to investigate the water condensation on surfaces. Here we use thermally controlled AFM (TC-AFM) [17] , [18] to directly investigate both the structure and in situ dynamics of water condensation on mica (hydrophilic surface) in both the hydrophobic–hydrophilic interface (graphene and mica) and the hydrophilic–hydrophilic interface (MoS 2 and mica). By carefully monitoring the whole dynamic water growth process, the water interaction within the hydrophobic–hydrophilic interface was investigated. Further, molecular dynamics (MD) simulation was used to study the individual water molecular absorption process, and a rational growth model for water condensation was discussed. Our study is particularly relevant to water biological compatibility because differences in water condensation phases may occur when it interacts with the hydrophobic or hydrophilic surfaces of biological molecules [19] . Experimental design overview With the aim of temperature-dependent investigation, a heating-up and cooling-down process was designed to in situ monitor how the water diffusion and condensation traversed between the atmosphere and the interface ( Fig. 1a ). Under ambient conditions (25 °C; relative humidity (RH) ~35%), freshly cleaved mica substrate is hydrophilic and thus will inevitably absorb a heterogeneous water film (whole layer or islands of water molecules) with a thickness depending on the ambient RH [14] , [20] . Given this default water layer on the mica surface, graphene and MoS 2 sheets were then carefully transferred onto mica through mechanical exfoliation ( Fig. 1b ) [21] , [22] . To eliminate the effect from the exfoliation tap, a so-called tap-free method was used in our study [13] , [21] . Localized by their optical contrast and Raman spectroscopy, a graphene sheet and a MoS 2 monolayer were selected, respectively ( Fig. 1c , left; and Supplementary Figs 1 and 2 ). Further characterization by AFM shows the well-defined single/bilayer graphene and single/bilayer MoS 2 ( Fig. 1c , right). There are many water plateaus on the MoS 2 sample, and with sample-to-sample variations such island-like plateaus can also be observed in graphene samples even via tape-free mechanical exfoliation ( Supplementary Fig. 3 ), in agreement with previous reports [11] , [14] , [16] . The plateaus show no obvious difference in phase contrast with the surrounding elevated areas ( Supplementary Fig. 4 ), which indicates that these plateau structures occurred initially under both graphene and MoS 2 sheets, which further confirmed the sandwich arrangement as shown in Fig. 1b [11] , [14] . 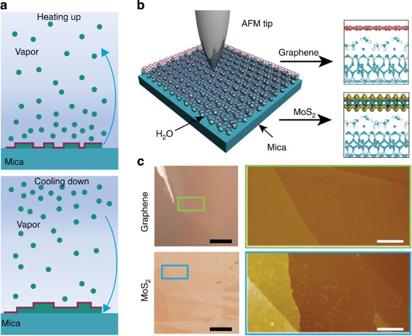Figure 1: Experiment design and microscopy image of as-prepared samples. (a) A heating-up and cooling-down process presented toin situmonitor the water diffusion and condensation that occurred between the atmosphere and the interface. (b) Schematic representation showing the experimental setup where a single-layer graphene or MoS2is used as an ideal template for studying the condensation of water vapour on mica under ambient conditions. The cartoon pictures present a clear sandwich structure, where water adlayers were trapped at the hydrophobic–hydrophilic interface (graphene and mica) and the hydrophilic–hydrophilic interface (MoS2and mica). (c) Optical images (left) and AFM images (right) of graphene and MoS2on mica surface, which present well-defined single/bilayer adlayers with underneath of water domains under ambient condition (RT, RH ~35%). Scale bars, 10 μm in the left images and 2 μm in the right images. Figure 1: Experiment design and microscopy image of as-prepared samples. ( a ) A heating-up and cooling-down process presented to in situ monitor the water diffusion and condensation that occurred between the atmosphere and the interface. ( b ) Schematic representation showing the experimental setup where a single-layer graphene or MoS 2 is used as an ideal template for studying the condensation of water vapour on mica under ambient conditions. The cartoon pictures present a clear sandwich structure, where water adlayers were trapped at the hydrophobic–hydrophilic interface (graphene and mica) and the hydrophilic–hydrophilic interface (MoS 2 and mica). ( c ) Optical images (left) and AFM images (right) of graphene and MoS 2 on mica surface, which present well-defined single/bilayer adlayers with underneath of water domains under ambient condition (RT, RH ~35%). Scale bars, 10 μm in the left images and 2 μm in the right images. Full size image Water diffusion The above well-prepared samples were first heated up to 100 °C for the dewetting process. Fractals growth was clearly observed in the graphene–water–mica system; meanwhile the fractals appeared to be continuous across single-layer–bilayer borders, as shown in the Fig. 2a . Corresponding with the red dashed line in Fig. 2a , the line profile provided a quantitative measurement of the depth of the fractals, 3.7±0.2 Å, which is in agreement with the height of a single monolayer of ice –I h [11] . We provide a control experiment to evaluate the bare mica without graphene coating while changing the temperature from RT to 100 °C, and no fractal-like pattern is generated (data not shown here). It is revealed that those fractal-like patterns were due to water diffusion rather than due to the formation of microstructures such as domains or ripples by the ion migration from the mica. These interesting phenomena encouraged us to perform a detailed research on the dewetting process at each selected temperature. Our state-of-the-art TC-AFM setup with controlled temperature resolution of 1 °C makes this case realizable. The graphene–water–mica sandwich system was in situ imaged by AFM upon a gradual temperature increase from RT to 100 °C. The heating rate was set at 2 °C min −1 , and upon each step of 10 °C the temperature was maintained for 30 min while capturing an AFM image. 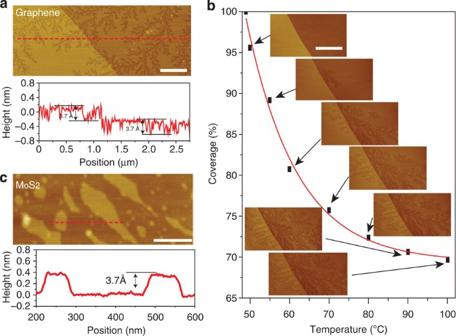Figure 2: Visualization of the fractal structures growth with increasing temperature. (a) AFM image and height line profile of the graphene sheet are presented to show the water diffusion at high temperature (T=100 °C). Scale bar, 500 nm. (b)In situAFM images of graphene–water–mica structures were recorded from RT to 100 °C in steps of 10 °C. The growth dynamics curve was characterized by the water coverage as a function of temperature, and the red line is an exponential fit. The same dewetting experiment was also performed for the MoS2samples. Scale bar, 2 μm. (c) AFM image and height line profile of the MoS2sheet show the same water monolayers covered by graphene. However, no obvious changes with the temperature increase from RT to 100 °C occurred for the MoS2–water–mica system (Supplementary Fig. 4). Scale bar, 100 nm. Figure 2b shows that no noticeable change was observed below 40 °C, whereas a small depression grew into fractal structures when the temperature reached 50 °C. Further increase in temperature led the fractals to grow much faster, which slowed down when the temperature reached 80 °C. The quantitative water coverage, θ , defined as , where A f is the fractal and A 0 the whole scanning area, was calculated and is plotted in Fig. 2b . An extremely similar result was reported previously, where the ambient RH was controlled to reversibly dewet the water film on the mica surface covered by graphene [14] . It means that increasing the temperature has a similar effect as reducing RH, and thus also leads to dewet the water film confined between graphene and mica referring to the diffusion-limited aggregation growth mechanism (three-dimensional (3D) image and illustrated model in Supplementary Fig. 5 ) [14] . The same dewetting experiments have also been performed on the MoS 2 system, in which totally different phenomena occurred. The water plateaus were still present but without any fractals ( Fig. 2b ). From the line profile, it is known that these water plateaus are also ~3.7 Å, which should also be a single monolayer of ice –I h . We demonstrate that the same water monolayer has been covered by both graphene and MoS 2 ; however, with increasing temperature the water diffusing could only occur at graphene/mica. Figure 2: Visualization of the fractal structures growth with increasing temperature. ( a ) AFM image and height line profile of the graphene sheet are presented to show the water diffusion at high temperature ( T =100 °C). Scale bar, 500 nm. ( b ) In situ AFM images of graphene–water–mica structures were recorded from RT to 100 °C in steps of 10 °C. The growth dynamics curve was characterized by the water coverage as a function of temperature, and the red line is an exponential fit. The same dewetting experiment was also performed for the MoS 2 samples. Scale bar, 2 μm. ( c ) AFM image and height line profile of the MoS 2 sheet show the same water monolayers covered by graphene. However, no obvious changes with the temperature increase from RT to 100 °C occurred for the MoS 2 –water–mica system ( Supplementary Fig. 4 ). Scale bar, 100 nm. Full size image Frank-van der Merwe growth for second water adlayer W ith the knowledge of the above dewetting process, the pertinent rewetting process is further performed to investigate the water condensation process. TC-AFM was used to cool down the sample from 100 °C to RT. Interestingly, island-like plateaus were observed after about an hour of cooling at the graphene/mica interface, where the original fractals (named as the first water adlayer) still revealed no change ( Fig. 3aI ). In particular, the plateaus exhibited no obvious difference in phase contrast with the surrounding elevated areas, which may indicate that these plateau structures occurred under the graphene sheets ( Supplementary Fig. 4 ) [11] , [14] . Furthermore, at low coverage, the isolated island-like plateaus grew independently, whereas upon high water coverage they eventually coalesced into a continuous adlayer ( Fig. 3aII–VIII , time interval from Fig. 3aI of 18, 27, 36, 45, 54, 63 and 72 min, respectively). The same method, as shown in Fig. 2b , was used to plot the plateaus’ coverage tendency with time ( Fig. 3b ). For quantitative plateau coverage, μ is defined as , where A p is the plateaus’ area and A 0 is the whole scanning area. With appropriate fitting, the growth of plateaus also followed an exponential function. 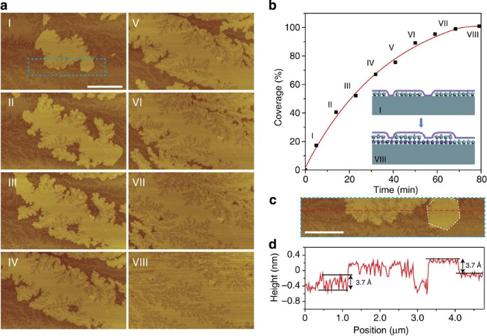Figure 3: Visualizing the growth of the second water adlayer. (a)In situAFM images (I–VIII) of the second water adlayer growth during water condensation with time. Scale bar, 2 μm. (b) Dynamics growth of the second water adlayer as a function of time; the red line is an exponential fit. The illustration in the inset depicts the whole growth of a second water adlayer with Frank-van der Merwe (FM) mode. (c) Zoom-in of the AFM image of the plateau structures shown inFig. 3aI. Scale bar, 1 μm. (d) Height line profile corresponding to the red dashed line inFig. 3c. Figure 3c is the zoom-in AFM image of Fig. 3aI revealing the nature of these plateaus. Interestingly, a hexagon boundary marked with a white dashed line clearly appeared. In addition, another work [20] , which was performed without graphene coating, also present the similar hexagon shape on mica via scanning polarization force microscopy. At the same time, other experimental and theoretical works have also clearly pointed out a close match between the lattice constant of the water adlayer and the underlying mica substrate [11] , [23] , [24] , [25] , [26] . To further reveal the relative orientation of the water adlayer, the atomic structures are recorded by high-resolution AFM. The hexagonal shape of water adlayers was aligned with the axes of supported mica crystal instead of the graphene or MoS 2 coating layers ( Supplementary Fig. 6 ). Besides, as shown with the line profile ( Fig. 3d ), these islands were 3.7±0.2 Å in height relative to the first adlayer thickness, which is again in good agreement with the layer thickness of ice –I h . Collectively, one can conclude that these plateaus were also ice-like structures, which were named as the second ice-like water adlayer. The results confirm that two confined layers of ice-like water adlayers can be observed at RT, and, at the same time, the whole dynamic growth process was directly visualized to prove that the second ice-like water adlayer was directly stacked on top of the first water adlayer. It is in good agreement with other previous experiments and theoretical simulations. [4] , [11] , [16] , [27] Furthermore, the mechanically exfoliated graphene sheet was proved to be impermeable to small molecules [13] , [28] , which suggests that the water molecule from the second water adlayer diffused through the edges of the graphene/mica interface. Besides, the same experiment has been performed for the MoS 2 –water–mica system. Not surprisingly, no obvious changes occurred during the cooling-down process, which present the same phenomenon as the heating-up process. The intrinsic mechanism will be discussed later. Figure 3: Visualizing the growth of the second water adlayer. ( a ) In situ AFM images (I–VIII) of the second water adlayer growth during water condensation with time. Scale bar, 2 μm. ( b ) Dynamics growth of the second water adlayer as a function of time; the red line is an exponential fit. The illustration in the inset depicts the whole growth of a second water adlayer with Frank-van der Merwe (FM) mode. ( c ) Zoom-in of the AFM image of the plateau structures shown in Fig. 3aI . Scale bar, 1 μm. ( d ) Height line profile corresponding to the red dashed line in Fig. 3c . Full size image Volmer–Weber growth for third water adlayer Surprisingly, a third and even thicker water droplet has also been occasionally captured during the water condensation process. 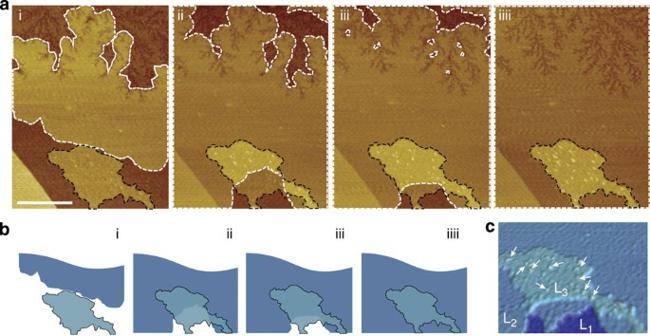Figure 4: Visualizing the growth of the third island-like water adlayer. (a)In situmulti-AFM images of another sample after naturally cooling down from 100 °C, where the third water adlayer (black dashed line) appears beside the second water adlayer (white dashed line). Scale bar, 1 μm. (b) Subarea modelling dynamic process (from i to iiii) to illustrate the approaching pathway of the second water adlayer vis-à-vis the third water adlayer. (c) 3D AFM image for all three water adlayers (L1, the first water adlayer, L2, the second water adlayer; and L3, the third water adlayer). Figure 4a shows an in situ multi-AFM image of the graphene–water–mica sample during the cooling-down process from 100 °C, where the third water adlayer (black dashed line) appears beside the second water adlayer (white dashed line) as the stacked-up model. At the same time, it is worth noticing that the original fractals (named as the first water adlayer) also underwent no change as presented above. Further, it was observed that the second water adlayer grew larger and larger, and gradually covered the entire scanning area after ~40 min ( Fig. 4ai–iiii ). In order to clearly show this process, the subarea dynamic modelling process is illustrated in Fig. 4b (from i to iiii), demonstrating the approaching pathway of the second water adlayer vis-à-vis the third water adlayer. Time-lag imaging was performed to check sufficient growth of the third water adlayer. However, the third water adlayer (black dashed line) underwent no change, while, instead, protruding water domains were observed as indicated by the white arrows in Fig. 4c . The protruding water domains appeared roundish and were thought to be liquid-like (named as water droplets). Following 24 h of additional incubation at RT, a thicker third water adlayer appeared, and, importantly, it still remained island-like rather than as an integrated film ( Supplementary Fig. 7 ). At the same time, the coarse fractal patterns formed by the first water adlayer disappeared, which meant that extra water molecules could fill into the coarse fractal space. These third ice-like water adlayers were for the first time directly visualized experimentally on the hydrophilic mica substrate with assistance of the hydrophobic graphene, which has been theoretically predicted by the previous report [25] . Meanwhile, the whole water condensation process, from monolayer to triple layer and then to water droplets, was also clearly shown here. The SK growth model has been used to describe the whole water condensation process at the hydrophobic–hydrophilic interface in a following discussion. Figure 4: Visualizing the growth of the third island-like water adlayer. ( a ) In situ multi-AFM images of another sample after naturally cooling down from 100 °C, where the third water adlayer (black dashed line) appears beside the second water adlayer (white dashed line). Scale bar, 1 μm. ( b ) Subarea modelling dynamic process (from i to iiii) to illustrate the approaching pathway of the second water adlayer vis-à-vis the third water adlayer. ( c ) 3D AFM image for all three water adlayers (L 1 , the first water adlayer, L 2 , the second water adlayer; and L 3 , the third water adlayer). Full size image In the water diffusion process, it was surprising that the epitaxial growth of the second water adlayer occurred between the first water adlayer and mica substrate while observing the second water adlayer growth. It means that unusual adsorption of the first water adlayer on the hydrophobic graphene occurred, which was known to only exist at cryogenic temperature (between 100 and 140 K; ref. 24 ). Generally, the binding energy of the water to the hydrophilic substrate is stronger compared with that to the hydrophobic substrate. However, the lack of bonding to the hydrophobic substrate will induce stratification in the water near the interface, which provides the possibility to grow quasi-2D crystalline on the hydrophobic substrate, such as graphene [23] , [24] , [27] , [29] . Even though the detailed mechanism is still unclear, the vicinity of the first water adlayer into graphene instead of the mica surface is probably because of the surface defects on the graphene surface after annealing [11] . Besides, the hydrophobic graphene surface will also guide the water diffusion along the zigzag direction of the C–C bond [26] . Furthermore, previous studies have agreed that no dangling hydrogen bonds are found in the first ice –I h adlayer on mica or the graphene surface [11] , [24] , [25] . On the basis of the above analysis, the second and even the third water adlayers should be epitaxially formed at almost zero pressure between mica and the first ice –I h adlayer interface. Further, MD simulation was used to study the water adsorption process on mica as shown in Fig. 5a,b . The effect of graphene coating on the structure of the water adlayer was also studied. The adsorption process slowed down when there were ~275 water molecules on the upper surface of the mica, corresponding to the full first water adlayer ( Supplementary Fig. 8 ). The tendency of the adsorption curve revealed by the simulation is consistent with our experiment result as shown in Fig. 3b . The structure of the water adlayer is characterized by the distribution of the water oxygen atom along the z -direction (normal of mica plane). There were three sublayers ( Fig. 5a at z =1.7 Å (peak 1, P1), z =2.7 Å (peak 2, P2) and z =3.6 Å (peak 3, P3)) in the first water layer, which also agreed with the suggestion by Odelius et al. [30] ( Supplementary Figs 8 and 9 ). Hence, our simulation result could reliably reflect the real water adsorption process to some extent. The structure of the water adlayer after graphene coating was further studied. Specifically, there were 10 systems with the following number of water molecules: N =150, 200, 230, 250, 275, 300, 320, 350, 375 and 400, respectively. Compared with the case in the absence of graphene coating, the layering structure of the adsorbed water became more ordered after the graphene was placed on top of it. The distributions corresponding to two water layers (first layer: 1.1 Å< z <4.6 Å and second layer: 4.6 Å< z <8.1 Å) became sharper. In the cases of N =150 and 200, the distribution of the binding site 3 (P3) vanished; in the case of N =250, the distribution of the second layer (P4) shrank while the distribution of binding site 3 (P3) enhanced; in the case of N =300, the distribution of the second layer (P4) became distinct rather than the tail. According to the layering structure revealed by water density distribution in Fig. 5a,b , we calculated the number of water molecules that belonged to the first and the second layer separately. The maximum number of water molecules in the first layer, N first , was 250 (in the case of N =275), only 87% of the value of the ideally fully occupied water layer, that is, 288. In addition, the second layer began to appear when N first = N =230. The second water layer began to appear before the formation of the fully occupied first water layer. More surprisingly, N first considerably decreased from 250 to 231 as N increases from 275 to 350. The result suggests that there are at least 20 water molecules that translocate from the first layer to the second layer during the growth of the water adlayer. The simulation results also suggested that the first water layer in our experiment was not the ordinary water layer that occurred during the water condensation process. In addition, the result is well consistent with the experimental observation about the unusual adsorption of the first ice-like water adlayer on the hydrophobic graphene at RT, which was used to be known to only exist at cryogenic temperature. 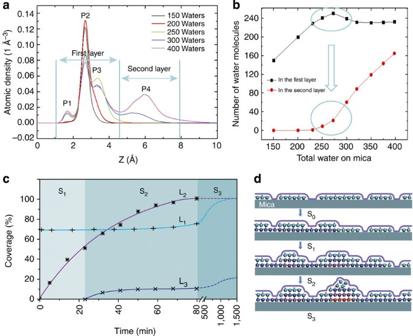Figure 5: MD simulation and moulding water growth with the SK model. (a) Density distributions of adsorbed water up to 400 molecules on mica with graphene coating. In the case of 250 water molecules, the distribution corresponding to the second layer (P4) was absent, whereas the distribution of binding site 3 (P3) was enhanced. With more water molecule adsorption, the distribution of the second layer (P4) becomes distinct rather than the tail in the case of 300 water molecules. (b) Number of water molecules in the first two layers during the adsorption process. The value ofNfirstdecreases as theNincreases from 275 to 350, which suggests the translocation of water molecules from the first layer to the second layer. (c) Full map of the dynamic water growth for all three water adlayers (L1, L2and L3). The growth can be easily divided into three stages: stage one, S1: the rapid growth of the second water layer with the third water layer absent; stage two, S2: the continued growth of the second water layer with slow rate till the entire layer, meanwhile the starting growth of the third layer; and stage three, S3: the third layer growth with little progress, with the fractal patterns gradually disappearing. (d) Schematic diagram for more impressive imaging of the whole water adlayer growth process, followed by the SK growth model. Figure 5: MD simulation and moulding water growth with the SK model. ( a ) Density distributions of adsorbed water up to 400 molecules on mica with graphene coating. In the case of 250 water molecules, the distribution corresponding to the second layer (P4) was absent, whereas the distribution of binding site 3 (P3) was enhanced. With more water molecule adsorption, the distribution of the second layer (P4) becomes distinct rather than the tail in the case of 300 water molecules. ( b ) Number of water molecules in the first two layers during the adsorption process. The value of N first decreases as the N increases from 275 to 350, which suggests the translocation of water molecules from the first layer to the second layer. ( c ) Full map of the dynamic water growth for all three water adlayers (L 1 , L 2 and L 3 ). The growth can be easily divided into three stages: stage one, S 1 : the rapid growth of the second water layer with the third water layer absent; stage two, S 2 : the continued growth of the second water layer with slow rate till the entire layer, meanwhile the starting growth of the third layer; and stage three, S 3 : the third layer growth with little progress, with the fractal patterns gradually disappearing. ( d ) Schematic diagram for more impressive imaging of the whole water adlayer growth process, followed by the SK growth model. Full size image Combining all the experimental observations and MD simulation, we try to present the dynamic plot of water growth on mica with graphene coating ( Fig. 5c ; three water adlayers L 1 , L 2 and L 3 , as indicated in Fig. 4c ). Overall, the growth stages can be clearly divided into four stages: stage zero (S 0 ), the initial single-layer ice-like water formation on the mica surface; stage one (S 1 ), the rapid growth of the second water layer epitaxially formed at almost zero pressure between mica and the first ice –I h adlayer interface, with the third water layer absent in the meanwhile; stage two (S 2 ), the continued growth of the second water at a slow rate until complete coverage, while the third layer appeared; stage three (S 3 ), the third layer growth with little progress between mica and the second ice –I h adlayer interface, but the fractal patterns were gradually disappearing owing to the further liquid-state water present, providing the basis for a general model of water growth ( Fig. 5d and Supplementary Fig. 10 ). For the previous reports, an FM growth model [31] was proposed to describe the water growth process [11] , [16] . However, the FM growth model is one of three distinct growth models. The initial water film growth follows an FM growth model, while, beyond this point, the water growth continues through the nucleation and coalescence of an island-like domain following a Volmer–Weber-type mechanism. [32] After a comprehensive evaluation, it was found that the SK growth model [33] lies between the Volmer–Weber and FM models, which is more appropriate to describe the whole water growth process in our experiment. Meanwhile, an ab initio MD study has demonstrated that, compared with the monolayer and t bilayer, slightly higher structural stability occurred on the water trilayer ewith the assistance of graphene [25] . In the natural water condensation process, the transition from flat water crystal to droplets is common. Within the hydrophobic–hydrophilic interface under ambient conditions, we were able to directly observe the SK growth process of water in good agreement with previous experiments at cryogenic temperatures [4] . Overall, both heating-up and cooling-down processes have clearly shown significant difference in the water diffusion between the hydrophobic and hydrophilic interfaces ( Fig. 6b,c ). Previous reports have agreed that muscovite mica (001) with K + cations will inevitably absorb a first epitaxial water adlayer. This first epitaxial water adlayer shows little motions owing to strong hydrogen bonds with the ion on the mica surface. With coating graphene or MoS 2 monolayer, the initial water adlayer presents more stability and less movability, especially with MoS 2 coating. The MoS 2 –water–mica system, in other words, the hydrophilic–hydrophilic interface, shows no obvious changes with the temperature increase from RT to 100 °C, as well as in the following cooling-down process. It demonstrated that water diffusing could only occur at graphene/mica, in other words, the hydrophobic–hydrophilic interface. These phenomena can be explained as follows: (1) Water molecules could be charge polarized, which in turn would bond to Mo and S atoms ( Fig. 6a ) [34] . Then, the water adlayers would be easily trapped in the MoS 2 and mica interface. (2) Stronger van der Waals force exists between the hydrophilic–hydrophilic interface (MoS 2 /mica) than between the hydrophobic–hydrophilic interface (graphene/mica), which can tightly seal the space between the MoS 2 and mica [16] . By contrast, water diffusing was observed to be disengaged at the hydrophobic–hydrophilic (graphene/mica) interface for the first water adlayer ( Fig. 6c ), which was further stacked by the second and third water adlayers. This direct visualization of water growth at the interface in this study may provide a valuable method for the study of condensed phase of water, and even shed light on the surface science studies of other small molecule adlayers at the solid interface. 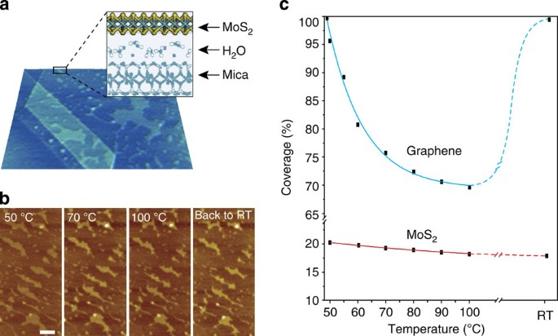Figure 6: Comparison of water behaviour at the MoS2and graphene surface. (a) Schematic representation showing the MoS2–water–mica ‘sandwich’ structure. (b)In situAFM images of MoS2–water–mica structures recorded in steps of 10 °C from RT to 100 °C, and then back to RT. It clearly shows that the MoS2–water–mica sandwich structure shows no obvious changes with the temperature increase, and at the same time, for the cooling-down process, there is also no obvious changes in the water adlayers. Scale bar, 100 nm. (c) The dynamic coverage of the first water adlayer under both graphene and MoS2coating is plotted, which demonstrates that water diffusing could not easily occur at the MoS2and mica interface compared with at the graphene and mica interface. Figure 6: Comparison of water behaviour at the MoS 2 and graphene surface. ( a ) Schematic representation showing the MoS 2 –water–mica ‘sandwich’ structure. ( b ) In situ AFM images of MoS 2 –water–mica structures recorded in steps of 10 °C from RT to 100 °C, and then back to RT. It clearly shows that the MoS 2 –water–mica sandwich structure shows no obvious changes with the temperature increase, and at the same time, for the cooling-down process, there is also no obvious changes in the water adlayers. Scale bar, 100 nm. ( c ) The dynamic coverage of the first water adlayer under both graphene and MoS 2 coating is plotted, which demonstrates that water diffusing could not easily occur at the MoS 2 and mica interface compared with at the graphene and mica interface. Full size image Preparation of graphene/MoS 2 samples The graphene/MoS 2 sheets were deposited by mechanical exfoliation of natural graphene/MoS 2 (Alfa Aesar, USA) onto the freshly cleaved muscovite mica substrate under ambient conditions (RT; RH ~35%). In order to avoid the effect from the exfoliation tape, a tape-free method [14] , [35] was followed for all the samples in our experiments. Graphene/MoS 2 sheets were located by their contrast under optical microscopy and were further confirmed by Raman and AFM characterization. Raman spectroscopy The Raman spectroscopy characterization was performed using micro-Raman spectroscopy (Renishaw inVia Raman Spectroscope, Sweden). The wavelength and power of the laser were set at 514 nm and 1.0 mW. A × 100 objective lens with numerical aperture=0.90 was used to focus the laser beam on the sample, which resulted in a laser spot of ~1.0 μm. AFM characterization The AFM data were acquired on a home-built TC-AFM (TC-AFM) based on a Multimode Nanoscope V (Bruker, Santa Barbara, USA). The scanner was equipped with an external heating element that offered a suitable platform for the thermally responsive experiment. Temperature variation was accomplished via a resistive heating stage (temperature range: RT to 250 °C and resolution: 0.1 °C). A cooling water fluid circuit refrigerates the piezo-scanner. Before the acquisition of every image, a dwell time of 5 min was allowed to equilibrate the temperature [17] . AFM image acquisition was carried out in tapping mode in air (probes: OMCL-AC160TS-C2, Olympus, Japan). The high-resolution AFM images were carried out under contact mode (probes: MLCT-F, Bruker). The AFM images were further analysed using SPIP software (Image Metrology, Denmark). The step height (0.34 nm) from double layer to single-layer graphene was used to calibrate the Z-piezo of AFM. MD simulation The box size for the simulation was 62.2 × 35.8 × 200 Å 3 , and the mica surface was composed of 48 unit cells, and the interaction of mica was described by the CLAFF force field [36] . There were 4,110 water molecules in the systems, and the TIP4P/2005 water model was used ( Supplementary Fig. 7 ). All the simulations were carried out in the isothermal–isobaric ensemble with 1 bar pressure and a temperature of 300 K. The total simulation time for water adsorption was 1,250 ns, and there were up to 400 water molecules adsorbed on the surface of the mica. How to cite this article: Song, J. et al. Evidence of Stranski–Krastanov growth at the initial stage of atmospheric water condensation. Nat. Commun. 5:4837 doi: 10.1038/ncomms5837 (2014).